Spin injection and detection in lanthanum- and niobium-doped SrTiO3using the Hanle technique There has been much interest in the injection and detection of spin-polarized carriers in semiconductors for the purposes of developing novel spintronic devices. Here we report the electrical injection and detection of spin-polarized carriers into Nb-doped strontium titanate single crystals and La-doped strontium titanate epitaxial thin films using MgO tunnel barriers and the three-terminal Hanle technique. Spin lifetimes of up to ~100 ps are measured at room temperature and vary little as the temperature is decreased to low temperatures. However, the mobility of the strontium titanate has a strong temperature dependence. This behaviour and the carrier doping dependence of the spin lifetime suggest that the spin lifetime is limited by spin-dependent scattering at the MgO/strontium titanate interfaces, perhaps related to the formation of doping induced Ti 3+ . Our results reveal a severe limitation of the three-terminal Hanle technique for measuring spin lifetimes within the interior of the subject material. Interest in oxide thin films and heterostructures has been stimulated by potential nano-electronic applications especially as functional oxides can be integrated with mainstream Si-based semiconductor electronic platforms [1] , [2] , [3] . Over the past decade, the properties of SrTiO 3 (strontium titanate, STO) interfaces and thin films, in particular, have attracted much attention, stimulated especially by the discovery of a high mobility two-dimensional electron gas (2DEG) at the interface between STO and several other perovskites [1] , [2] , [4] , as well as in La-doped STO thin films [5] . The possibility of spin injection and accumulation in STO films and at the 2DEG interface between LaAlO 3 /STO [6] promises novel spin-based devices. Here we report the successful injection of spin-polarized electrons and their accumulation in bulk Nb-doped STO substrates and La-doped STO thin films at temperatures as high as room temperature, as characterized via a three-terminal Hanle measurement [7] , [8] , [9] , [10] , [11] . The current flows from an ohmic contact (Al/Ta/Au) through the STO and back through a ferromagnetic (FM) electrode that acts as the spin injector/detector (MgO/CoFe/Ta/Au), as shown in Fig. 1a . The spin-dependent chemical potential is characterized by the voltage between another ohmic contact as the reference and the FM injector/detector. The spin injection through a tunnelling barrier (2 nm MgO) yields a net spin accumulation in the STO conduction band, which is described by the difference of the spin up and spin down electrochemical potentials (Δ μ = μ ↑ −μ ↓ ), as shown in Fig. 1b . The spin accumulation is measured as Δ V = γ Δ μ /2 e , where γ is the tunnelling spin polarization of the in-plane magnetized FM spin injector/detector (CoFe). The spin accumulation is detected by applying an out-of-plane magnetic field ( B z ) perpendicular to the electron spin direction ( Fig. 1c ), which causes the spins to precess in-plane, resulting in a decrease of the measured spin accumulation due to spin dephasing. The spin precesses at the Larmor frequency defined by = gμ B B / ħ , where g is the g -factor ( g =2 for STO) [5] , μ B is the Bohr magneton, and ħ is the reduced Planck’s constant. 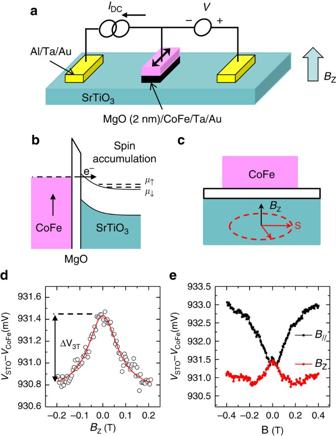Figure 1: Device geometry and three-terminal Hanle measurement. (a) Device geometry: the tunnelling contact is formed from 2 nm MgO/CoFe/Ta/Au. (b) Tunnelling spin injection: the spin-dependent chemical potential is split for spin-up and spin-down carriers. (c) Hanle spin measurement schematic. (d) Hanle measurement on a Nb (0.7 wt%) -doped SrTiO3single crystal (Nb:STO1) with a carrier doping of 1.2 × 1019cm−3(T=10 K,IDC=500 μA). The arrow indicates the Hanle spin voltage signal (ΔV3T). (e) Inverted Hanle and Hanle curves measured with an in-plane (B//) and an out-of-plane magnetic field (Bz), respectively, (T=10 K,IDC=500 μA). Figure 1: Device geometry and three-terminal Hanle measurement. ( a ) Device geometry: the tunnelling contact is formed from 2 nm MgO/CoFe/Ta/Au. ( b ) Tunnelling spin injection: the spin-dependent chemical potential is split for spin-up and spin-down carriers. ( c ) Hanle spin measurement schematic. ( d ) Hanle measurement on a Nb (0.7 wt%) -doped SrTiO 3 single crystal (Nb:STO1) with a carrier doping of 1.2 × 10 19 cm −3 ( T =10 K, I DC =500 μA). The arrow indicates the Hanle spin voltage signal (Δ V 3T ). ( e ) Inverted Hanle and Hanle curves measured with an in-plane ( B // ) and an out-of-plane magnetic field ( B z ), respectively, ( T =10 K, I DC =500 μA). Full size image Spin injection into Nb-doped STO using the Hanle technique The Hanle curve measures the voltage between the STO and CoFe as a function of out-of-plane magnetic field. A typical Hanle curve is shown in Fig. 1d , which is measured on a Nb-doped STO sample (labelled Nb:STO1; Nb doping: 0.7 wt%, 1.2 × 10 19 cm −3 ) at 10 K with a DC current of 500 μA. The spin lifetime ( τ ) is about 75 ps, as obtained by fitting the measured results with the equation Δ V ( B z )=Δ V (0)/(1+( τ ) 2 ) (red curve in Fig. 1d ). The measured spin signal Δ V 3 T is characterized by the difference between the voltages measured without magnetic field and when the magnetic field is large enough to cause the net spin accumulation to approach zero. In contrast to the nonlocal Hanle measurement [12] , [13] , the measured spin lifetime directly probes the spin properties in the STO beneath the CoFe injector/detector. Owing to spin relaxation induced by random magnetic fields from, for example, the roughness of CoFe film, a lower bound of the spin lifetime is found [14] . To confirm the authenticity of the measured spin signal, we measure the inverted Hanle effect by applying an in-plane magnetic field to enhance the component of the effective field along the direction of the spin polarization of the injected electrons ( Fig. 1e ). At high magnetic fields, the Hanle and inverted Hanle curves match each other (see Supplementary Fig. S1 ), which confirms the success of spin injection and detection in STO [10] . Whereas spin injection corresponds to electrons flowing from the CoFe electrode into the STO (positive DC current), spin extraction refers to the opposite flow of electrons from STO into the CoFe (negative DC current). The latter process also gives rise to spin accumulation in the STO [15] as majority electrons preferentially flow from STO to CoFe, thereby leaving behind minority spin-polarized carriers in the STO. Thus, the difference between the majority and minority spin chemical potentials will be negative. 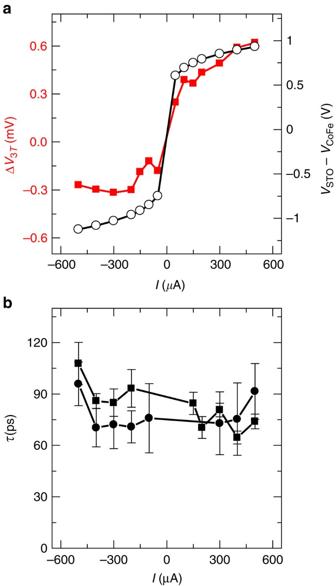Figure 2: Bias dependence of the Hanle signal. (a) Spin voltage signal ΔV3Tas a function of injection current (red squares), and, current-voltage characteristic of the CoFe/MgO/SrTiO3tunnel injector (black circles) for the Nb:STO1 sample at 10 K. (b) Bias dependence of the spin lifetime measured at 10 K on two Nb (0.7 wt%) doped SrTiO3single crystals (black squares for Nb:STO1 and black circles for Nb:STO2) with the same carrier doping of 1.2 × 1019cm−3. Error bars correspond to 95% confidence levels. Figure 2a compares the DC bias current dependence of the spin signal with that of the voltage drop across the tunnel barrier for bulk Nb-doped STO (labelled Nb:STO1). At positive DC bias (spin injection), the spin signal is higher than that for negative DC bias (spin extraction), indicating a higher spin accumulation in the former case. This behaviour is likely related to the bias dependence of the electronic structure and/or the bias dependence of the spin injection/detection efficiency [16] . The bias dependence of the spin lifetime for this same sample was studied at 10 K, as summarized in Fig. 2b . The spin lifetime is ~100 ps and depends only weakly on the bias current. To confirm this result, a second Nb-doped STO sample (labelled Nb:STO2) with nominally the same doping concentration (0.7 wt%, 1.2 × 10 19 cm −3 ) as that of Nb:STO1 was also studied at 10 K. The bias dependence of the spin lifetime for these two samples, shown in Fig. 2b , are very similar. Figure 2: Bias dependence of the Hanle signal. ( a ) Spin voltage signal Δ V 3T as a function of injection current (red squares), and, current-voltage characteristic of the CoFe/MgO/SrTiO 3 tunnel injector (black circles) for the Nb:STO1 sample at 10 K. ( b ) Bias dependence of the spin lifetime measured at 10 K on two Nb (0.7 wt%) doped SrTiO 3 single crystals (black squares for Nb:STO1 and black circles for Nb:STO2) with the same carrier doping of 1.2 × 10 19 cm −3 . Error bars correspond to 95% confidence levels. Full size image Temperature dependence of the spin signals The temperature dependence of the Hanle curves measured on Nb:STO1 for spin injection (500 μA) and spin extraction (−500 μA) are shown in Fig. 3a , respectively. The asymmetry of the spin injection and extraction persists up to room temperature. At room temperature, the spin signals are ~0.3 and ~−0.1 mV for 500 μA and −500 μA bias currents, respectively. The successful electrical spin injection and accumulation at room temperature augurs well for possible future applications of oxide spintronics. A summary of the spin signals as a function of temperature are plotted in Fig. 3c . The spin voltages vary from ~0.1 to ~0.7 mV and the corresponding spin resistance-area products, R s × A , where A is the area of the contact (125 × 170 μm 2 ), are between 6 and 40 kΩ μm 2 . We note that these are significantly higher than theoretical values calculated from our measured spin diffusion lengths that we estimate vary from ~0.01 to 0.5 kΩ μm 2 . Such a discrepancy has previously been observed in Hanle studies of spin injection into various semiconductors but its origin is poorly understood [17] . One of these mechanisms attributes the high R s × A values (at a GaAs/ Al 2 O 3 interface) [18] to a two-step tunnelling mechanism via localized states. Such states could be formed at the Ti 3+ magnetic centres in our devices. 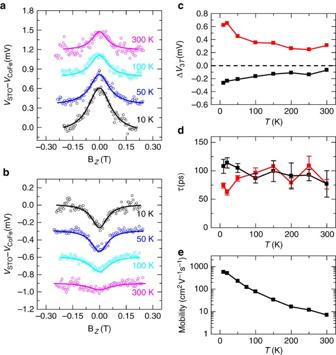Figure 3: Temperature dependence of the Hanle signal. (a,b) Hanle curves for Nb-doped SrTiO3(Nb:STO1 sample) at various temperatures for positive and negative bias currents of 500 μA. Temperature dependence of (c) spin voltage signal (red squares forIDC=500 μA and black squares forIDC=−500 μA), (d) spin lifetime (red squares forIDC=500 μA and black squares forIDC=−500 μA; error bars correspond to 95% confidence levels), and (e) mobility for the same sample. Figure 3: Temperature dependence of the Hanle signal. ( a , b ) Hanle curves for Nb-doped SrTiO 3 (Nb:STO1 sample) at various temperatures for positive and negative bias currents of 500 μA. Temperature dependence of ( c ) spin voltage signal (red squares for I DC =500 μA and black squares for I DC =−500 μA), ( d ) spin lifetime (red squares for I DC =500 μA and black squares for I DC =−500 μA; error bars correspond to 95% confidence levels), and ( e ) mobility for the same sample. Full size image Temperature dependence of the spin lifetime The summary of the spin lifetimes as a function of temperature are plotted in Fig. 3c . Although the spin lifetimes show little variation as a function of temperature, it is very interesting that the mobility, by contrast, exhibits a very strong temperature dependence, as shown in Fig. 3e . Indeed, the mobility in the Nb:STO1 sample increases by about a hundred-fold from room temperature to 10 K. Spin injection into La-doped STO High quality, epitaxial, stoichiometric La-doped STO films with high mobilities have been grown recently by oxide molecular beam epitaxy [5] . Here we focus on two different samples with carrier concentrations of 2.9 × 10 19 and 6.0 × 10 19 cm −3 as determined by Hall bar measurements. For the first sample with the lower dopant concentration, the Hanle spin signal can be detected up to ~200 K. The spin lifetime is ~50 ps and shows both a weak bias dependence as well as a weak temperature dependence, as summarized in Fig. 4a , respectively. For the sample with a higher dopant concentration, the Hanle spin signal can be detected up to ~100 K. The spin lifetime is found to be ~20 ps and is much shorter compared with the first sample with the lower dopant concentration. These results are summarized in Fig. 4d . 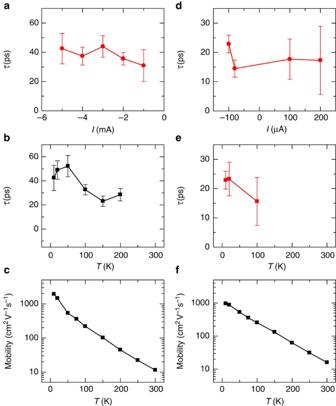Figure 4: Bias and temperature dependence of the Hanle signal for La-doped STO. Bias dependence of the spin lifetime at 10 K and temperature dependence of the spin lifetime and mobility measured for two La-doped SrTiO3films with doping concentrations of (a–c) 2.9 × 1019cm−3and (d–f) 6.0 × 1019cm−3.IDC=−5 mA inbandIDC=−100 μA inb. Error bars for spin lifetime values correspond to 95% confidence levels. Figure 4: Bias and temperature dependence of the Hanle signal for La-doped STO. Bias dependence of the spin lifetime at 10 K and temperature dependence of the spin lifetime and mobility measured for two La-doped SrTiO 3 films with doping concentrations of ( a – c ) 2.9 × 10 19 cm −3 and ( d – f ) 6.0 × 10 19 cm −3 . I DC =−5 mA in b and I DC =−100 μA in b . Error bars for spin lifetime values correspond to 95% confidence levels. Full size image An important observation is that in all of our samples the spin lifetime shows little variation with temperature whereas, by contrast, the mobility exhibits a strong temperature dependence ( Fig. 4c ). This observation strongly suggests that the spin lifetime is limited by spin-dependent scattering at the interfaces with the MgO tunnel barrier. Specifically, we hypothesize that the interface scattering is likely related to the formation of Ti 3+ magnetic centres at the MgO/STO interface formed by chemical doping of Nb or La (ref. 19 ). Indeed, evidence for such scattering is found from the Kondo effect observed in 2DEGs formed at the surface of STO single crystals when electrolyte gated [20] , [21] and the observation of magnetism at the LAO/STO interface [22] , [23] , [24] , which have both been attributed to the formation of Ti 3+ magnetic centres [20] , [21] , [25] , [26] . The spin lifetimes measured at 10 K on the various samples discussed above are summarized in Fig. 5a as a function of bias voltage. The pink colour corresponds to a Nb doping level of 1.2 × 10 19 cm −3 , and the green and grey colours correspond to La-doping levels of 2.3 × 10 19 and 6.0 × 10 19 cm −3 , respectively. The dependence of the spin lifetime on the carrier density and mobility are shown in Fig. 5b , respectively, for data corresponding to a bias voltage of ~−0.8 V. The mobility of La-doped STO decreases with increasing carrier concentration due to increased ionic impurity scattering [5] , [27] . The higher mobility of the La doped as compared with the Nb-doped STO can be attributed to the very high structural quality of the STO films [5] . 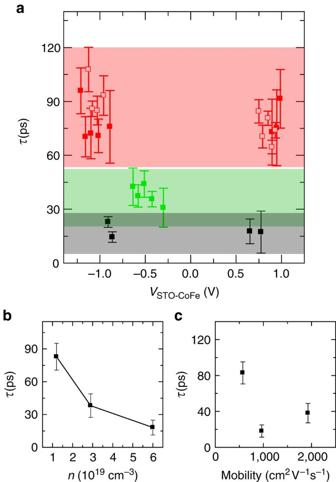Figure 5: Carrier doping dependence of the spin lifetime in STO. (a) Bias dependence of the spin lifetime measured for various dopant concentrations at 10 K (red squares/red open squares for Nb:STO1/Nb:STO2 with the same carrier doping of 1.2 × 1019cm−3, green squares for La:STO with the carrier doping of 2.9 × 1019cm−3and black squares for La:STO with the carrier doping of 6.0 × 1019cm−3). Spin lifetime as a function of (b) carrier density and (c) mobility measured at 10 K. Error bars correspond to 95% confidence levels. Figure 5: Carrier doping dependence of the spin lifetime in STO. ( a ) Bias dependence of the spin lifetime measured for various dopant concentrations at 10 K (red squares/red open squares for Nb:STO1/Nb:STO2 with the same carrier doping of 1.2 × 10 19 cm −3 , green squares for La:STO with the carrier doping of 2.9 × 10 19 cm −3 and black squares for La:STO with the carrier doping of 6.0 × 10 19 cm −3 ). Spin lifetime as a function of ( b ) carrier density and ( c ) mobility measured at 10 K. Error bars correspond to 95% confidence levels. Full size image Of considerable interest, the spin lifetime decreases systematically with increasing dopant concentration ( Fig. 5 ). We suggest that the decrease is due to a corresponding increase in the number of magnetic centres at the STO/MgO interface. Indeed previous X-ray photoemission spectroscopy studies on Nb- and La-doped STO [19] show that the Nb and La dopants have valence states of Nb 5+ and La 3+ , respectively, which gives rise to Ti 3+ centres, and that the concentration of Ti 3+ scales with the dopant concentration. As Ti 3+ has a magnetic moment, we hypothesize that the spin lifetime is limited by scattering from the Ti 3+ located at or near the MgO/STO interfaces. We note that longer spin lifetimes in Nb-doped STO as compared with La-doped STO may also be attributed to a difference in spin-orbit coupling constants resulting from the smaller atomic number of Nb. As mentioned earlier, the inverted Hanle and Hanle curves overlap each other at a magnetic field of ~2 T: this is the field required to saturate the magnetization of the CoFe electrode, as seen, for example, in measurements of the anisotropic magnetoresistance of CoFe (see Supplementary Fig. S1c ). When the moment of the CoFe electrode is oriented along the field (above 2 T) there can be no Hanle or inverted Hanle effect. Thus, our experiments are limited to fields below 2 T. However, very large magnetic fields are required to saturate the paramagnetic moments on the Ti 3+ ( s =1/2) centres. For example, at 10 K, assuming the magnetic moments follow a Brillouin function with no exchange between the moments, a field of 2 T will orient the moments to only 13% of their saturation moment. When the temperature is higher the moments will be even less ordered by the magnetic fields in which we can observe a Hanle or inverted Hanle effect. Thus, we conclude that the Ti 3+ moments will be fluctuating significantly for all the temperatures and magnetic fields in which we observe the Hanle or inverted Hanle effects. We conclude that it is magnetic scattering from these randomly oriented moments that depolarize the injected carriers and that this mechanism is weakly dependent on temperature and therefore consistent with the weak temperature dependence that we find in our Hanle and inverted Hanle data (see Supplementary Fig. S3 ). In summary, spin injection and spin detection in doped STO bulk crystals and thin films has been achieved up to room temperature using MgO tunnel spin injectors. The spin lifetimes are about 100 ps, which are similar to conventional semiconductors such as GaAs and Si with similar carrier densities and doping levels using the same Hanle technique [8] , [10] , [11] , [18] . Interestingly, we find that the spin lifetime has a very weak temperature dependence even though the carrier mobility in the doped STO samples has, by contrast, a very strong temperature dependence. We thus conclude that the spin lifetime is limited by spin-dependent scattering from magnetic centres at the STO/MgO interfaces, which we attribute to Ti 3+ formed as a result of the La and Nb doping. Our results show that the Hanle technique to measure the spin polarization of carriers injected via a tunnel contact is strongly influenced by the formation of these contacts and thus may not be a reliable indicator of the spin lifetime within the interior of the STO itself. Device fabrication Nb-doped SrTiO 3 (0.7 wt%) substrates were obtained from Princeton Scientific Corporation. La-doped SrTiO 3 films were epitaxially grown on undoped SrTiO 3 (001) substrates using oxide molecular beam epitaxy as reported in detail elsewhere [5] . The Nb:STO substrates and La:STO films were cleaned using the following procedure: wash in methanol in an ultrasonic bath for 10 min, followed by a distilled water wash in an ultrasonic bath for 10 min, a dip in hydrogen peroxide for 30 s, and finally a distilled water rinse. Then the samples were heated in a furnace at either 1,000 °C (Nb:STO) or 900 °C (La:STO) for ~90 min in a pure oxygen environment that results in the formation of atomically flat surfaces, which we confirmed by atomic force microscopy [28] . The spin injection/accumulation devices were fabricated using shadow masks in an ultra high vacuum sputtering system. The tunnelling contact is formed from 2 nm MgO, 10 nm CoFe, 5 nm Ta and 20 nm Au and has an area of 125 × 170 μm 2 . The ohmic contact is formed from 10 nm Al, 5 nm Ta and 20 nm Au. The RMS roughness averaged over an area of 10 × 10 μm 2 was ~0.16 nm for the as prepared Nb:STO1 sample, and was increased only slightly to ~0.29 nm after a 2-nm-thick MgO tunnel barrier was deposited on top of the same sample. Electrical measurement The electrical measurements were performed in a PPMS (Quantum Design) system. The mobility, carrier density and resistivity were characterized using van der Pauw and Hall bar geometries. The carrier density shows little temperature dependence for both Nb:STO single crystals (see Supplementary Fig. S2 ) and La:STO films [5] . The carrier density values used here are those measured at room temperature. Contact characterization The temperature dependent I–V characteristics of a typical contact (CoFe/MgO/Nb:STO1) are characterized by the three-terminal method and shown in Fig. 6 . The I–V characteristics are highly non-linear and the contact resistance shows a modest increase as the temperature decreases, which are two important characteristics of tunnelling contacts [29] . 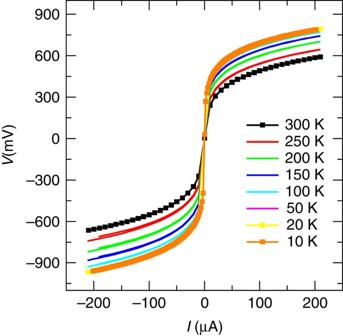Figure 6 Temperature dependent I–V characteristics of a typical contact on a Nb doped STO device. Figure 6 Temperature dependent I–V characteristics of a typical contact on a Nb doped STO device. Full size image How to cite this article: Han, W. et al. Spin injection and detection in lanthanum- and niobium-doped SrTiO 3 using the Hanle technique. Nat. Commun. 4:2134 doi: 10.1038/ncomms3134 (2013).